Hygro-responsive membranes for effective oil–water separation There is a critical need for new energy-efficient solutions to separate oil–water mixtures, especially those stabilized by surfactants. Traditional membrane-based separation technologies are energy-intensive and limited, either by fouling or by the inability of a single membrane to separate all types of oil–water mixtures. Here we report membranes with hygro-responsive surfaces, which are both superhydrophilic and superoleophobic, in air and under water. Our membranes can separate, for the first time, a range of different oil–water mixtures in a single-unit operation, with >99.9% separation efficiency, by using the difference in capillary forces acting on the two phases. Our separation methodology is solely gravity-driven and consequently is expected to be highly energy-efficient. We anticipate that our separation methodology will have numerous applications, including the clean-up of oil spills, wastewater treatment, fuel purification and the separation of commercially relevant emulsions. Recent events including the Deepwater Horizon oil spill in the Gulf of Mexico have highlighted the difficulty of effective oil–water separation. Efficient, cost-effective processes for oil–water separation, especially in the presence of dispersants (or surfactants), are greatly desired [1] . Surfactant-stabilized mixtures of oil and water are classified [2] , in terms of the diameter ( d ) of the dispersed phase, as free oil and water if d >150 μm, a dispersion if 20 μm ≤ d ≤ 150 μm, or an emulsion if d <20 μm. Conventional gravity separators and skimming techniques are incapable of separating emulsions [2] . Membrane-based technologies are attractive for demulsification (the conversion of an emulsion to a free oil–water mixture) because they are relatively energy-efficient, cost-effective, and are applicable across a wide range of industrial effluents [2] . However, for complete oil–water separation, demulsification is typically followed by either gravity separation or skimming. Membranes are typically classified as either hydrophobic or hydrophilic [3] , [4] , [5] , [6] , [7] , [8] , [9] , [10] . Their wettability by oil is often not specified because, in most cases, such membranes are oleophilic, that is, their contact angle with oil is <90°. Hydrophobic (or superhydrophobic [9] , [10] , [11] ) and oleophilic membranes are typically used in energy-intensive cross-flow filtration systems [3] , [6] , [7] because they are unsuitable for gravity-driven oil–water separation. This is because water naturally settles below oil and against the membrane owing to its higher density, forming a barrier layer that prevents oil permeation. Hydrophobic and oleophilic membranes are also easily fouled by oil during demulsification [6] , [7] . Although conventional hydrophilic membranes can be used for gravity-driven demulsification, and are more resistant to fouling [2] , they are unsuitable for the separation of free oil–water mixtures or water-in-oil emulsions because both oil and water can easily permeate through them (see Supplementary Fig. S1 and Supplementary Discussion ). As many as three different phases (oil, oil-in-water or water-in-oil emulsion and water) may co-exist in oil–water mixtures [12] , [13] . To effect the gravity-driven separation of all types of oil–water mixtures in a single step, the ideal membrane is expected to be hydrophilic (or superhydrophilic [14] ) and oleophobic (or superoleophobic [15] ), both in air and when submerged in water. However, a membrane that is oleophobic in air typically loses its oleophobicity under water, and vice versa [16] , [17] . Most surfaces that are superoleophobic (displaying apparent contact angles for oil of θ * oil >150°) are also superhydrophobic [15] , [18] , [19] . This is due to the higher surface tension of water, which results in the respective Young's contact angles [20] satisfying θ water > θ oil . A few studies [14] , [21] , [22] , [23] , [24] , [25] , [26] have reported surfaces where θ water < θ oil , which was achieved by using specific interactions between water and the substrate to lower the solid–liquid interfacial tension ( γ sl ). However, with two exceptions [14] , [25] all such surfaces were oleophilic. The systematic design of membranes for oil–water separation requires the parameterization of two important physical characteristics: surface porosity, which affects the rate of permeation of one phase (for example water) through the membrane, and breakthrough pressure ( P breakthrough ), the maximum pressure difference across the membrane below which the membrane prevents the permeation of the second phase (for example oil). Recent work [15] , [18] , [19] , [27] , [28] , [29] , [30] has explained how 're-entrant surface texture', in conjunction with surface chemistry and roughness, can be used to design superoleophobic surfaces. We have previously discussed the spacing ratio, D *, which is a dimensionless measure of surface porosity [19] . For substrates possessing a cylindrical texture, such as those considered here, D *=( R + D )/ R , where R is the cylinder radius and 2 D is the intercylinder spacing. Higher values of D * indicate higher porosity and, therefore, a higher permeation rate for the contacting liquid. We also discussed the robustness factor [19] , A *, which is the ratio of P breakthrough and a reference pressure, P ref =2 γ lv / l cap . Here is the capillary length for the liquid, γ lv is the liquid surface tension, ρ is the liquid density and g is the acceleration due to gravity. The reference pressure is approximately the minimum possible pressure that may be applied to a membrane by commonly occurring liquid droplets or puddles [19] . As a result, any membrane with A *≤1 for a given liquid cannot prevent liquid permeation, whereas values of A * 1 imply a high resistance to liquid permeation. For surfaces possessing a cylindrical texture, the robustness factor is given by [19] , [28] Recently, we reported a gravity-assisted, electric field-driven methodology for separation of oil–water emulsions in a single-unit operation [31] . However, that methodology requires continuous application of a very high voltage and is limited to separation of a few millilitres of emulsions. Guided by the design parameters discussed above, in this paper we develop novel membranes with hygro-responsive surfaces [30] , which are both superhydrophilic ( θ * water ≈0°) and superoleophobic ( θ * oil >150°) both in air and under water. Our membranes can separate, for the first time, several litres of oil–water mixtures, including surfactant-stabilized emulsions, solely using gravity, in a single-unit operation, with >99.9% separation efficiency, by using the difference in capillary forces acting on the two phases. Our separation methodology is solely gravity-driven and consequently is expected to be highly energy-efficient. We demonstrate the separation of several litres of oil–water mixtures using a scaled-up apparatus. We also demonstrate continuous separation of oil–water emulsions for over 100 h without a decrease in flux. 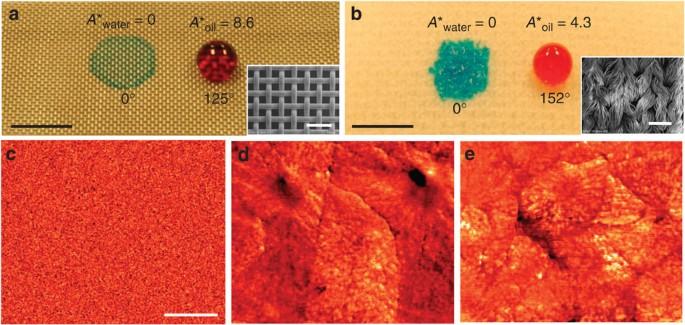Figure 1: Wetting behaviour of water and oil. (a,b), Droplets of water (dyed blue) and rapeseed oil (dyed red) on stainless steel mesh 100 (a) and polyester fabric (b). Both surfaces have been dip-coated with a 20 wt% fluorodecyl POSS+x-PEGDA blend. Scale bars, 5 mm. Insets, morphologies of the respective dip-coated mesh and fabric surfaces. Scale bars, 500 μm. (c–e) AFM phase images of surfaces coated with x-PEGDA (c), a 10 wt% fluorodecyl POSS+x-PEGDA blend (d) and a 20 wt% fluorodecyl POSS+x-PEGDA blend (e). The phase angle ranges are 0°–115° (c), 0°–25° (d) and 0°–21° (e). Scale bar, 2 μm. Wetting behaviour of water and oil Figure 1a,b show the wetting behaviour of water ( γ lv =72.1 mN m −1 ) and rapeseed oil ( γ lv =35.7 mN m −1 ) on a stainless steel mesh 100 ( Fig. 1a , inset; Methods) and polyester fabric ( Fig. 1b , inset), each dip coated with a blend of 20 wt% fluorodecyl polyhedral oligomeric silsesquioxane (POSS) [15] and cross-linked poly(ethylene glycol) diacrylate (x-PEGDA; Methods). For a surface spin coated with a 20 wt% fluorodecyl POSS+x-PEGDA blend (solid surface energy γ sv =10.5 mN m −1 , see Supplementary Table S1 ), the advancing contact angle for rapeseed oil is θ oil,adv =88°. This yields A * oil values of 8.6 and 4.3 for rapeseed oil on the mesh and fabric membranes, respectively. Because D * fabric =6 is greater than D * mesh =2.2, the observed apparent advancing contact angle on the dip-coated fabric ( θ * oil,adv =152°) is higher than that on mesh 100 ( θ * oil,adv =125°). However, despite their low surface energies, both the fabric and the mesh membranes are readily permeated by water, with θ * water =0°. This is a direct consequence of the surface reconfiguration induced by the contacting water droplet, as discussed below. Figure 1: Wetting behaviour of water and oil. ( a , b ), Droplets of water (dyed blue) and rapeseed oil (dyed red) on stainless steel mesh 100 ( a ) and polyester fabric ( b ). Both surfaces have been dip-coated with a 20 wt% fluorodecyl POSS+x-PEGDA blend. Scale bars, 5 mm. Insets, morphologies of the respective dip-coated mesh and fabric surfaces. Scale bars, 500 μm. ( c – e ) AFM phase images of surfaces coated with x-PEGDA ( c ), a 10 wt% fluorodecyl POSS+x-PEGDA blend ( d ) and a 20 wt% fluorodecyl POSS+x-PEGDA blend ( e ). The phase angle ranges are 0°–115° ( c ), 0°–25° ( d ) and 0°–21° ( e ). Scale bar, 2 μm. Full size image Figure 1c–e shows atomic force microscope (AFM) phase images of x-PEGDA and two fluorodecyl POSS+x-PEGDA blends in air. Although crystalline domains are absent on the neat x-PEGDA surface ( Fig. 1c ), the surfaces of both the 10 wt% ( Fig. 1d ) and the 20 wt% ( Fig. 1e ) blends are completely covered with crystalline domains of fluorodecyl POSS. This indicates substantial surface segregation of the fluorodecyl POSS molecules, as may be expected owing to their extremely low surface energies [15] . This surface migration leads to a rapid decrease in both the dispersive ( γ d sv ) and the polar components ( γ p sv ) of the blend surface energy (see Supplementary Fig. S2 , Supplementary Table S1 and Supplementary Discussion ). 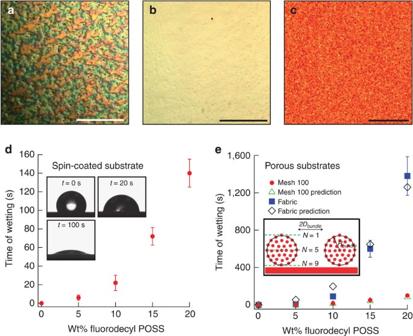Figure 2: Surface reconfiguration and ToW. (a,b) Optical microscopy images of a surface coated with a 20 wt% fluorodecyl POSS+x-PEGDA blend in air (a) and under water (b). Scale bars, 300 μm. (c)In situ, underwater AFM phase image of a surface coated with a 20 wt% fluorodecyl POSS+x-PEGDA. The phase angle range is 0°–112°. Scale bar, 2 μm. (d,e) ToW of water for spin-coated (d) and porous (e) substrates. Error bars, s.d.;n=5. Insets indshow the time-dependent decrease in contact angle for a water droplet. Inset ineis a schematic illustrating the two scales of texture (bundles and individual fibres) for the fabric. The ToW predictions for mesh 100 and fabric membranes closely match experimental measurements, as shown ine. Surface reconfiguration and time of wetting Figure 2a,b display optical images of spin-coated surfaces of 20 wt% fluorodecyl POSS+x-PEGDA, in air ( Fig. 2a ) and under water ( Fig. 2b ). In air, the surface is relatively rough, with several fluorodecyl POSS aggregates. However, under water, fluorodecyl POSS aggregates disappear to reveal a smoother surface that is indicative of surface reconfiguration ( Supplementary Movie 1 ). PEGDA chains reconfigure to increase their interfacial area with water and facilitate enthalpic gains through hydrogen bonding. Surface reconfiguration is further confirmed by the absence of large crystalline domains in the in situ , underwater AFM phase image ( Fig. 2c ). We conducted multiple water wetting–drying cycles and found that this surface reconfiguration is reversible (see Supplementary Fig. S3 and Supplementary Discussion ). Surface energy analysis of the wet surface suggests that it is equivalent to an x-PEGDA blend with ~0.4–1.5 wt% fluorodecyl POSS (see Supplementary Discussion ). Figure 2: Surface reconfiguration and ToW. ( a , b ) Optical microscopy images of a surface coated with a 20 wt% fluorodecyl POSS+x-PEGDA blend in air ( a ) and under water ( b ). Scale bars, 300 μm. ( c ) In situ , underwater AFM phase image of a surface coated with a 20 wt% fluorodecyl POSS+x-PEGDA. The phase angle range is 0°–112°. Scale bar, 2 μm. ( d , e ) ToW of water for spin-coated ( d ) and porous ( e ) substrates. Error bars, s.d. ; n =5. Insets in d show the time-dependent decrease in contact angle for a water droplet. Inset in e is a schematic illustrating the two scales of texture (bundles and individual fibres) for the fabric. The ToW predictions for mesh 100 and fabric membranes closely match experimental measurements, as shown in e . Full size image Addition of fluorodecyl POSS causes a systematic increase in the time required for surface reconfiguration, as is evident from the increased time of wetting (ToW) for water on spin-coated fluorodecyl POSS+x-PEGDA surfaces ( Fig. 2d ). This is likely due to a reduction in the initial interfacial area between PEGDA chains and the contacting water droplet with increasing fluorodecyl POSS concentration. We define ToW as the time required for the water contact angle on a surface to decrease from its initial value to 0°. We also measured ToW for water on the porous mesh and fabric membranes ( Fig. 2e ). On these surfaces, we define ToW as the time required for the water droplet to imbibe into the membrane. Membrane imbibition is not instantaneous for surfaces with reconfigurable chemistry. Rather, the water–air interface progressively penetrates into the surface texture and water permeates through the membrane once the robustness factor A * water ≤ 1. (If the liquid does not permeate through the membrane pores, the solid–liquid–air composite interface equilibrates at a location on the membrane where the local texture angle ( ψ ) is equal to the Young's contact angle, θ .) From equation (1), for mesh 100, A * water =1 when θ water =18°. Our ToW measurements on the dip-coated meshes match closely with the time required for θ water,adv to decrease from its initial value to 18° ( Fig. 2e ). The ToW for water on the dip-coated fabrics was found to be considerably higher than ToW on the meshes. This is because water has to progressively wet multiple fibres during imbibition. The fabrics used in this work have interwoven bundles of fibres ( Fig. 1b , inset). Each bundle contains several layers of smaller individual fibres that offer an additional length scale for air entrapment ( Fig. 2e , inset). From equation (1), for water on an individual fibre ( R fibre =5 μm, D fibre =20 μm), A * water =1 when θ water =7°. Thus, the ToW for water on each layer of the fibres should be equal to the time taken for θ water,adv to reach 7°, which is approximately equal to the ToW for water on spin-coated substrates. Assuming N layers of individual fibres, the ToW for water on the fabric surface should be N times the ToW for water on the spin-coated surface. Fitting the experimental data with this N layer model yields a best fit for N= 9, which seems to be a reasonable estimate, based on Fig. 1b , inset. Capillary force-based separation Very few reports on membrane separation [25] , [32] , [33] and microfluidics [34] , [35] have used the difference in capillary forces acting on the two phases as the primary mechanism to separate emulsions or dispersions. We call this methodology capillary force-based separation (CFS). In CFS, the wetting phase permeates through the membrane, whereas the non-wetting phase is retained. From equation (1), the breakthrough pressure required to force the non-wetting phase through a membrane already saturated by the wetting phase is Here γ 12 is the interfacial tension between the wetting phase and the non-wetting phase, and θ is the contact angle of the non-wetting phase on the solid surface, both of which are completely immersed in the wetting phase. When pressure P applied < P breakthrough is applied, only the wetting phase permeates through the membrane. We use CFS in this work because it combines both demulsification and separation into a single-unit operation, it provides a very high-quality permeate and it is inherently self-repairing [34] . For a CFS-based system to work effectively, it is necessary that the wetting phase contact the membrane. There are several techniques to achieve this goal: gravity-driven (if the wetting phase has a higher density than the non-wetting phase), electrostatic (if the wetting phase is a polar liquid) [36] , forced convection [3] , [6] , [7] , etc. In this work, we demonstrate a proof-of-concept prototype that solely utilizes gravity to engender separation of various oil–water mixtures. 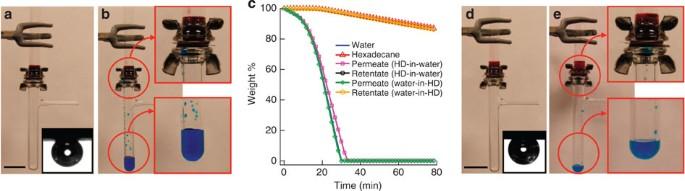Figure 3: Batch separation of oil-in-water and water-in-oil emulsions. (a) Separation apparatus with a 50:50 v:v hexadecane-in-water emulsion above the membrane. Inset, hexadecane droplet on a surface spin-coated with a 20 wt% fluorodecyl POSS+x-PEGDA blend, submerged in water containing dissolved SDS (1 mg ml−1). (b) Water-rich permeate passes through the membrane whereas hexadecane-rich retentate is retained. (c) TGA data for the permeates and the retentates. HD, hexadecane. (d) Apparatus with a 30:70 v:v water-in-hexadecane emulsion above the membrane. Inset, hexadecane droplet on a surface spin coated with a 20 wt% fluorodecyl POSS+x-PEGDA blend, submerged in water containing dissolved PS80 (1 mg ml−1). (e) Water-rich permeate passes through the membrane whereas hexadecane-rich retentate is retained. Water is dyed blue and hexadecane is dyed red. Scale bars, 2 cm. Separation of oil-in-water emulsions Figure 3a,b shows solely gravity-driven CFS of a hexadecane-in-water emulsion (50 vol% hexadecane; Methods) stabilized using SDS (hydrophilic–lipophilic balance, HLB=40). The hexadecane droplet size distribution (see Supplementary Fig. S4 and Supplementary Discussion ) indicates that the greatest number fraction of droplet diameters is in the range of 10–20 μm. The separation apparatus consists of a mesh 400 (2 D =37.5 μm), dip-coated with a 20 wt% fluorodecyl POSS+x-PEGDA blend and sandwiched between two vertical glass tubes. We used the superhydrophilic and oleophobic meshes here as they are available in a range of different pore sizes, allowing us to systematically vary the membrane porosity. Our superhydrophilic and superoleophobic fabrics show a similar performance. The emulsion is added to the upper tube ( Fig. 3a ). Once water in the emulsion contacts the membrane, the surface starts to reconfigure. Within minutes, the water-rich permeate passes through the membrane while the hexadecane-rich retentate is retained above the membrane ( Fig. 3b ). Membrane oleophobicity under water is critical for the separation of hexadecane-in-water emulsions ( Fig. 3a , inset). Optical image analysis indicates that the membrane removes virtually all hexadecane droplets exceeding 40 μm in diameter (see Supplementary Fig. S5 and Supplementary Discussion ). Thermogravimetric analyses (TGA; Fig. 3c ), transmittance and density measurements (see Supplementary Fig. S6 and Supplementary Discussion ) indicate that the permeate contains ~0.1 wt% hexadecane, whereas the retentate contains ~0.1 wt% water. Additional experiments showed that we can similarly separate, with >99% efficiency, hexadecane-in-water emulsions containing 10 vol% and 30 vol% hexadecane. We also conducted experiments with hexadecane-in-water emulsions containing salt (sodium chloride). As with the non-saline emulsions, we could separate saline emulsions with >99% efficiency. Figure 3: Batch separation of oil-in-water and water-in-oil emulsions. ( a ) Separation apparatus with a 50:50 v:v hexadecane-in-water emulsion above the membrane. Inset, hexadecane droplet on a surface spin-coated with a 20 wt% fluorodecyl POSS+x-PEGDA blend, submerged in water containing dissolved SDS (1 mg ml −1 ). ( b ) Water-rich permeate passes through the membrane whereas hexadecane-rich retentate is retained. ( c ) TGA data for the permeates and the retentates. HD, hexadecane. ( d ) Apparatus with a 30:70 v:v water-in-hexadecane emulsion above the membrane. Inset, hexadecane droplet on a surface spin coated with a 20 wt% fluorodecyl POSS+x-PEGDA blend, submerged in water containing dissolved PS80 (1 mg ml −1 ). ( e ) Water-rich permeate passes through the membrane whereas hexadecane-rich retentate is retained. Water is dyed blue and hexadecane is dyed red. Scale bars, 2 cm. Full size image Separation of water-in-oil emulsions Figure 3d,e shows the solely gravity-driven CFS of a water-in-oil emulsion (30 vol% water; Methods) stabilized using Polysorbate80 (PS80; HLB=15). The apparatus is the same as that used for the separation of oil-in-water emulsions. The emulsion is added to the upper tube ( Fig. 3d ). Once water droplets within the emulsion contact the membrane, the surface starts to reconfigure. Before the breakthrough of the water-rich permeate, hexadecane is retained above the membrane because of membrane oleophobicity in air. After surface reconfiguration, the water-rich permeate passes through the membrane while the hexadecane-rich retentate is retained above the membrane ( Fig. 3e ). During the permeation of the water-rich permeate, the hexadecane-rich retentate is retained above the membrane because of membrane oleophobicity under water. Membrane oleophobicity, both in air and under water, is critical for separating water-in-hexadecane emulsions. TGA ( Fig. 3c ), transmittance and density measurements (see Supplementary Fig. S6 and Supplementary Discussion ) indicate that the permeate contains ~0.1 wt% hexadecane, whereas the retentate contains ~0.1 wt% water. Additional experiments showed that we can similarly separate, with >99% efficiency, water-in-hexadecane emulsions containing 10 vol% and 20 vol% water. Further, we can also similarly separate span80 (HLB=4.3) stabilized water-in-hexadecane emulsions containing 10, 20 and 30 vol% water, with >99% efficiency. Our analysis also indicates that after separation, the surfactant fractionates into both the water-rich and the hexadecane-rich phases, depending upon its relative solubility in each phase (see Supplementary Fig. S7 and Supplementary Discussion ). 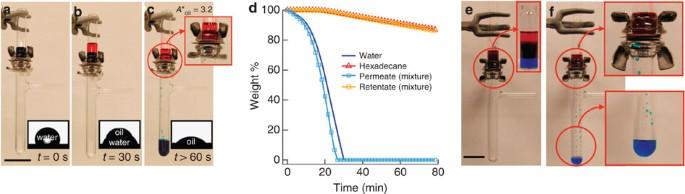Figure 4: Batch separation of free oil and water and four component mixtures. (a) Separation apparatus with water above the membrane. (b) Rapeseed oil is added above water. (c) Water permeates through the membrane whereas rapeseed oil is retained. Insets, water droplet on a surface spin-coated with a 20 wt% fluorodecyl POSS+x-PEGDA blend, rapeseed oil droplet on top of the water droplet, rapeseed oil droplet on the reconfigured surface. (d) TGA data for the permeate and the retentate. HD, hexadecane. (e) Apparatus with the four-component mixture above the membrane. Inset, larger quantity of feed in a glass vial, depicting the presence of different phases. (f) Water-rich permeate passes through the membrane whereas hexadecane-rich retentate is retained. Water is dyed blue, hexadecane and rapeseed oil are dyed red. Scale bars, 2 cm. Separation of free oil and water Figure 4a–c show the solely gravity-driven CFS of free rapeseed oil and water using a mesh 100 (2 D= 138 μm) coated with a 20 wt% fluorodecyl POSS+x-PEGDA blend. Water is added to the upper tube ( Fig. 4a ) immediately followed by rapeseed oil ( Fig. 4b ). The corresponding insets in Fig. 4a,b show a drop of water placed on a spin-coated surface of 20 wt% fluorodecyl POSS+x-PEGDA, and a drop of rapeseed oil immediately placed on top of the drop of water, respectively. Upon surface reconfiguration, water permeates through the membrane, while rapeseed oil is retained above the membrane ( Fig. 4c ). On a spin-coated 20 wt% fluorodecyl POSS+x-PEGDA surface, previously wet by water, a drop of rapeseed oil displays a contact angle of θ oil,adv =45° ( Fig. 4c , inset (ii)). Thus, for rapeseed oil on the membrane, the robustness factor A * oil =3.2. Consequently, rapeseed oil is retained above the membrane. A video illustrating the nearly complete separation of free oil and water is provided as Supplementary Movie 2 . As illustrated in the video, water permeates through the membrane at A * water =1.25. The experimentally measured flux of water through the membrane (mesh 100; 2 D =138 μm), Q water ≈43,200 l m −2 h −1 . This is significantly lower than the flux of the water (μ~1 mPa s), Q water =509,000 l m −2 h −1 , predicted using the Hagen–Poiseuille relation [37] . This is because the number of pores through which water is flowing at any given time (so-called 'active pores') in CFS can be significantly lower (~1−10%) than the actual number of pores [35] . Comparing the measured and the predicted fluxes, we estimate that ~8.5% of the total pores are active during the separation of free oil and water. Figure 4: Batch separation of free oil and water and four component mixtures. ( a ) Separation apparatus with water above the membrane. ( b ) Rapeseed oil is added above water. ( c ) Water permeates through the membrane whereas rapeseed oil is retained. Insets, water droplet on a surface spin-coated with a 20 wt% fluorodecyl POSS+x-PEGDA blend, rapeseed oil droplet on top of the water droplet, rapeseed oil droplet on the reconfigured surface. ( d ) TGA data for the permeate and the retentate. HD, hexadecane. ( e ) Apparatus with the four-component mixture above the membrane. Inset, larger quantity of feed in a glass vial, depicting the presence of different phases. ( f ) Water-rich permeate passes through the membrane whereas hexadecane-rich retentate is retained. Water is dyed blue, hexadecane and rapeseed oil are dyed red. Scale bars, 2 cm. Full size image Separation of four-component mixtures Figure 4e,f show the separation of a mixture containing four components: water, hexadecane, a 30:70 v:v water-in-hexadecane emulsion and a 50:50 v:v hexadecane-in-water emulsion. Again, mesh 400 dip coated with a 20 wt% fluorodecyl POSS+x-PEGDA blend separated this mixture into highly pure constituents, that is, a permeate containing ~0.1 wt% hexadecane and a retentate containing ~0.1 wt% water, as confirmed by TGA ( Fig. 4d ). To our knowledge, this is the first ever report of solely gravity-driven separation of surfactant-stabilized emulsions and their mixtures into highly pure constituents. Furthermore, the dip-coating-based membrane fabrication process is easy to scale up, and we have developed an apparatus to separate several litres of oil–water mixtures ( Supplementary Movie 3 ). As illustrated in the video, separation occurs even if the non-wetting phase (oil) contacts the dry membrane before the wetting phase. Breakthrough height For the separation apparatus shown in Figs 3 and 4 the maximum height of the liquid column before the oil phase permeates through the membrane ( h breakthrough ) can be obtained using equation (1) when the membrane is in air or equation (2) when the membrane is submerged under water. Note that P breakthrough = ρgh breakthrough . For free oil and water separation, θ oil,adv =45°, γ lv =35.7 mN m −1 and h breakthrough is predicted to be 1.3 cm ( P breakthrough =117 Pa) using equation (1). For the SDS-stabilized 50:50 v:v hexadecane-in-water emulsion, θ oil,adv =120° ( Fig. 3a , inset), γ 12 =4.0 mN m −1 and h breakthrough is predicted to be 2.3 cm ( P breakthrough =198 Pa) using equation (2). For water-in-oil emulsions, h breakthrough should be predicted using equation (1) before the breakthrough of the water-rich permeate and using equation (2) during the permeation of the water-rich permeate. The lower value of the two predicted breakthrough heights limits the operating height. For the PS80-stabilized 30:70 v:v water-in-hexadecane emulsion, before the breakthrough of the water-rich permeate, θ oil,adv =70°, γ lv =24.9 mN m −1 and h breakthrough is predicted to be 6.3 cm ( P breakthrough =519 Pa) using equation (1). For the same emulsion, during the permeation of the water-rich permeate, θ oil,adv =125° ( Fig. 3d , inset), γ 12 =3.7 mN m −1 and h breakthrough is predicted to be 2.4 cm ( P breakthrough =198 Pa). Consequently, the operating height during the water-in-hexadecane emulsion separation is limited by h breakthrough during the permeation of the water-rich permeate. Indeed, these predicted values of h breakthrough closely match experimentally measured values of 1.3 cm, 2 cm and 2.2 cm for the free oil and water, hexadecane-in-water emulsion and water-in-hexadecane emulsion separation, respectively. In the above analysis, we estimated the surface tension of hexadecane and the hexadecane–water interfacial tension, in the presence of surfactants, using the capillary-rise method [37] and the Fowkes [38] relationship (see Supplementary Discussion ). To ensure CFS, we used an operating height h < h breakthrough in all our separation operations. Continuous separation of oil–water emulsions In the separation apparatus design discussed above, oil accumulates above the membrane over time and will eventually break through once the operating height > h breakthrough . Therefore, we developed a continuous oil–water separation apparatus ( Fig. 5a ), with two CFS-based operations in parallel, using a superhydrophilic and oleophobic membrane at the bottom and a hydrophobic and oleophilic membrane on the side wall. Using this apparatus, we achieved continuous, solely gravity-driven CFS of oil–water emulsions ( Supplementary Movie 4 ). TGA ( Fig. 5b ) indicates that the water-rich permeate contains ~0.1 wt% hexadecane and that the hexadecane-rich permeate contains ~0.1 wt% water, which is the limit of detection using TGA. Karl Fischer analysis indicates that the hexadecane-rich permeate contains ~25±8 p.p.m. water, which is comparable to the solubility of water in hexadecane (~30 p.p.m. at 25 °C) (see Supplementary Discussion ). Analysis of the hexadecane-rich permeate also indicates that at least 99.8% of water droplets with diameter <20 μm are removed during separation (see Supplementary Fig. S8 and Supplementary Discussion ). Thus, it is clear that the membrane allows for the removal of dispersed-phase droplets that are considerably smaller than the membrane pore size (2 D =37.5 μm). To our knowledge, this is the first demonstration of continuous, solely gravity-driven CFS of surfactant-stabilized emulsions into highly pure constituents. 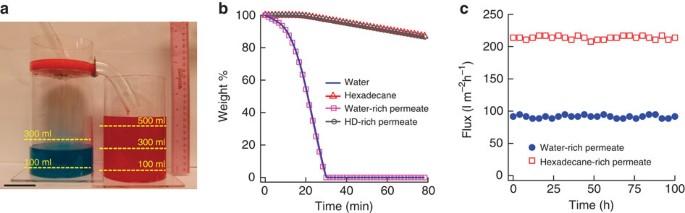Figure 5: Continuous separation of water-in-oil emulsions. (a) A scaled-up apparatus used for the continuous separation of 30:70 v:v water-in-hexadecane emulsions stabilized by polysorbate 80. The superhydrophilic and oleophobic mesh 400 was prepared by dip coating with a 20 wt% fluorodecyl POSS+x-PEGDA blend, whereas the hydrophobic and oleophilic mesh 400 was prepared by dip coating with Desmopan9370 (γsv=35.6 mN m−1; seeSupplementary Table S1andSupplementary Discussion). During continuous separation, water-rich permeate continuously passes through the superhydrophilic and oleophobic membrane, whereas hexadecane-rich permeate continuously passes through the hydrophobic and oleophilic membrane. Water is dyed blue and hexadecane is dyed red. Scale bar, 5 cm. (b) TGA data for both the permeates. (c) Measured fluxes for both the permeates as a function of time. Figure 5: Continuous separation of water-in-oil emulsions. ( a ) A scaled-up apparatus used for the continuous separation of 30:70 v:v water-in-hexadecane emulsions stabilized by polysorbate 80. The superhydrophilic and oleophobic mesh 400 was prepared by dip coating with a 20 wt% fluorodecyl POSS+x-PEGDA blend, whereas the hydrophobic and oleophilic mesh 400 was prepared by dip coating with Desmopan9370 ( γ sv =35.6 mN m −1 ; see Supplementary Table S1 and Supplementary Discussion ). During continuous separation, water-rich permeate continuously passes through the superhydrophilic and oleophobic membrane, whereas hexadecane-rich permeate continuously passes through the hydrophobic and oleophilic membrane. Water is dyed blue and hexadecane is dyed red. Scale bar, 5 cm. ( b ) TGA data for both the permeates. ( c ) Measured fluxes for both the permeates as a function of time. Full size image Fluxes of water-rich and hexadecane-rich permeates through the membranes were measured to be 90 and 210 l m −2 h −1 , respectively. These values are comparable to those reported in previous work on membrane separation under externally applied pressures [3] , [4] , [6] , [7] , [39] , [40] . Furthermore, in intermittent stop-and-go operation, the fluxes did not decrease over a period of 100 h ( Fig. 5c and Supplementary Table S2 ), indicating that the membranes are highly resistant to fouling by oil. Membrane wettability, and the considerably larger pore sizes of the membranes used here, compared with those used traditionally [3] , [5] , [7] , [8] , are expected to be two major contributing factors towards the observed resistance to fouling. The flux of the water-rich permeate during continuous separation of water-in-oil emulsions is limited by the sedimentation velocity of the water droplets. On the basis of this understanding, we predicted the flux to be Q water ≈83 l m −2 h −1 (see Supplementary Discussion ), which closely matches experimental results. However, as the pore size decreases, according to the Hagen–Poiseuille relation, the allowable flux of the water-rich permeate through membrane decreases. We calculated that the flux predicted by the Hagen–Poiseuille relation equals the flux predicted by the sedimentation velocity of the water droplets when the membrane pore diameter is ~4.5 μm. Thus, for all pore diameters 2 D 4.5 μm, the flux of water-rich permeate is only limited by the sedimentation velocity and is independent of the pore diameter. Indeed, experimentally we obtained almost the same flux for water using both mesh 400 (2 D =37.5 μm) and mesh 500 (2 D =30.5 μm) during continuous separation. A membrane with a smaller pore diameter, such as mesh 500, has a higher value for P breakthrough and is therefore more resistant to pressure perturbations. In conclusion, we have developed novel membranes with hygro-responsive surfaces, which are both superhydrophilic and superoleophobic. These membranes are oleophobic both in air and when submerged under water. Consequently, CFS-based unit operations using these membranes can separate a range of different oil–water mixtures, with >99% efficiency. We have also engineered an apparatus that uses two CFS-based operations in parallel to achieve continuous, solely gravity-driven separation of oil–water emulsions, with a separation efficiency ≥ 99.9%. We anticipate that our separation methodology will have numerous applications, including the clean-up of oil spills, wastewater treatment, fuel purification and the separation of commercially relevant emulsions. Materials PEGDA with a number-average molecular mass of M n ≈700 Da and its cross-linker 2-hydroxy-2-methyl propiophenone (Darocur1173) were obtained from Sigma Aldrich. Tecnoflon BR9151 fluoroelastomer was obtained from Solvay Solexis. Desmopan9370 polyurethane was obtained from Bayer Material Science. 1H, 1H, 2H, 2H-heptadecafluorodecyl polyhedral oligomeric silsequioxane (fluorodecyl POSS) was synthesized as described elsewhere [15] . Asahiklin AK-225 solvent was obtained from Structure Probe, Inc. Rapeseed oil, hexadecane, tetrahydrofuran, methylene blue (blue dye), oil red-o (red dye), sodium dodecyl sulphate, polysorbate 80 and span 80 were obtained from Fisher Scientific. Stainless steel meshes of mesh size 100 ( R =56.5 μm, 2 D =138 μm, D *=2.2), 400 ( R =12.5 μm, 2 D =37.5 μm, D *=2.5), 500 ( R =10.2 μm, 2 D =30.5 μm, D *=2.5) were obtained from McMaster Carr. The mesh number refers to the number of openings per inch. The fabric Anticon 100 ( R bundle =150 μm, 2 D bundle =300 μm, R fibre =5 μm, 2 D fibre =20 μm; D *=6 as described elsewhere [28] ) was obtained from VWR. Silicon wafers were obtained from the clean room at the University of Michigan. Substrate preparation Solutions (100 mg ml −1 ) of PEGDA, Darocur1173 and fluorodecyl POSS were prepared in Asahiklin AK-225. The PEGDA:Darcour1173 ratio was 95:5 w:w. The fluorodecyl POSS concentrations studied were 0, 0.5, 1, 2, 5, 10, 15 and 20 wt%. Solutions (10 mg ml −1 ) of Desmopan were prepared in tetrahydrofuran. Small pieces of mesh and fabric (2×2 cm) were dip-coated in the desired solution for 10 min and dried with nitrogen gas at room temperature (~22 °C) for 5 min. The non-textured substrates (silicon wafers, 2×2 cm) were spin-coated using Speciality Coating Systems Spincoater G3P-8 for 30 s at 250–2,000 r.p.m. (0.7–44.7 g ). After dip coating or spin coating, the PEGDA-containing surfaces were cross-linked for 5 min using a UVP XX-40S ultra violet bench lamp (wavelength, 254 nm). The thickness of the dip-coated layer varied between 100 nm and 1 μm. Oil–water emulsions Hexadecane-in-water emulsions (10:90, 30:70 and 50:50 v:v) were prepared by mixing water and hexadecane using a stir bar (at 700–1,200 r.p.m., or 3.4 – 10.1 g ) with 0.1–0.5 mg of SDS per ml of emulsion, whereas 10:90, 20:80 and 30:70 v:v water-in-hexadecane emulsions were prepared with 0.1–0.3 mg of PS80 per ml of emulsion and 0.1–0.3 mg of span 80 per ml of emulsion. Over time, a small degree of demulsification was observed for some emulsions. We determined whether an emulsion is hexadecane-in-water or water-in-hexadecane by measuring the electrical resistance with a multimetre. A KDScientific KDS-200 syringe pump was used to deliver the feed emulsions during continuous separation. Contact angle measurement All measurements of contact angle (in air and under water) were conducted using a Ramé–Hart 200-F1 goniometer. All contact angles reported in this work were measured by advancing or receding a small volume of liquid (~2 μl) onto the surface using a 2-ml micrometre syringe (Gilmont). At least three measurements were performed on each substrate. The typical error in measurements was ±2°. Microscopy Tapping-mode atomic force microscopy was conducted in air and under water using a Veeco Innova Instrument. Veeco TESPA tips were used for imaging in air, and Veeco SNL-10C tips were used for imaging under water. The thickness of the spin-coated films was determined using an AFM line scan across a scratched location. To ensure conformal coating, scanning electron microscopy of the dip-coated surfaces was conducted using a Hitachi SU8000 at 5 kV. Optical microscopy of the dry and wet spin-coated surfaces was conducted using an Olympus BH-2 optical microscope. Separation efficiency and droplet size distribution The water content in both the hexadecane-rich phase and the water-rich phase after separation was measured using a Perkin Elmer Pyris 1 TGA. Approximately 50 mg of the sample was heated from room temperature to 105 °C at a rate of 5 °C per min, and the temperature was held constant at 105 °C for 60 min. Note that the boiling point of hexadecane is 287 °C. The loss in weight of water was used to estimate the purity of the water-rich phase. The loss in weight of the hexadecane-rich phase was compared with the loss in weight of the as-obtained hexadecane to estimate the purity of the hexadecane-rich phase. The water content in the hexadecane-rich phase was also determined by injecting samples ranging in volume from 10 μl to 0.6 ml into an EM Science AquaStar C3000 Titrator for coulometric Karl Fischer titration analysis (ASTM D6304). The transmittance of the feed emulsions and permeates was measured using a Cary 50 Bio ultra violet-Visible spectrophotometer. The size distribution of the dispersed phase with droplet sizes <1 μm was determined by dynamic light scattering using a Malvern Zetasizer Nano ZS instrument. How to cite this article: Kota, A. K. et al . Hygro-responsive membranes for effective oil–water separation. Nat. Commun. 3:1025 doi: 10.1038/2027 (2012).